PADI4 acts as a coactivator of Tal1 by counteracting repressive histone arginine methylation The transcription factor Tal1 is a critical activator or repressor of gene expression in hematopoiesis and leukaemia. The mechanism by which Tal1 differentially influences transcription of distinct genes is not fully understood. Here we show that Tal1 interacts with the peptidylarginine deiminase IV (PADI4). We demonstrate that PADI4 can act as an epigenetic coactivator through influencing H3R2me2a. At the Tal1/PADI4 target gene IL6ST the repressive H3R2me2a mark triggered by PRMT6 is counteracted by PADI4, which augments the active H3K4me3 mark and thus increases IL6ST expression. In contrast, at the CTCF promoter PADI4 acts as a repressor. We propose that the influence of PADI4 on IL6ST transcription plays a role in the control of IL6ST expression during lineage differentiation of hematopoietic stem/progenitor cells. These results open the possibility to pharmacologically influence Tal1 in leukaemia. The translocated in leukaemia 1 (Tal1; or stem cell leukaemia, Scl) transcription factor is essential for the generation of embryonic hematopoietic stem cells (HSCs). Tal1-deficient mice are embryonically lethal owing to the absence of hematopoiesis and to vascular defects [1] , [2] , [3] , [4] . In adult hematopoiesis, Tal1 plays a role in gene regulation and differentiation of monocytes and osteoclasts [5] , [6] , and at the megakaryocyte/erythrocyte branching point [7] , [8] , [9] , [10] . Tal1 also participates in the control of the balance between proliferation and differentiation during erythroid differentiation and influences adult HSC quiescence [11] , [12] . Furthermore, ectopic expression of Tal1 caused by chromosomal translocation is linked to T-cell acute lymphoblastic leukaemia [13] , [14] , [15] . Mouse models suggest that additional alterations in cofactors of Tal1, such as LMO2, facilitate manifestation of the leukemogenic potential of Tal1 [16] , [17] , [18] , [19] . Tal1 is a bHLH-class transcription factor, which binds to the DNA-recognition E-box motif CANNTG as a heterodimer with E-proteins such as HEB or E47. Tal1 acts in gene and cell-type-specific gene regulatory complexes containing the E2A proteins, GATA1, RUNX1, FLI1, LMO2, Ldb1, ETS1 and ETO2 (MTG16) [11] , [20] , [21] , [22] , [23] , [24] . Furthermore, Tal1 can interact with the histone modifying coactivator proteins CBP/P300, P/CAF [25] and the corepressor proteins Sin3a and LSD1 [26] , [27] , [28] . These interactions determine whether Tal1 acts as a repressor or an activator of gene expression. For this reason, knowledge of the distinctive association of Tal1 with epigenetic cofactors is crucial to the understanding of Tal1 function. Moreover, because histone-modifying enzymes are accessible to small-molecule inhibitors, identification of Tal1 interacting enzymes could uncover targets for a molecular therapy of Tal1-dependent leukaemias. The peptidylarginine deiminase IV (PADI4 or PAD4) converts arginine residues at histone tails to citrulline [29] . Citrullination can take place at unmodified or methylated arginines and counteracts arginine methylation by protein arginine methyltransferases (PRMTs) [30] , [31] , [32] , [33] , [34] . In vitro PADI4 can deiminate arginine residues at positions H3R2, H3R8, H3R17 and H3R26, and PADI4 has been demonstrated to prevent arginine methylation at position H3R17 by PRMT4 (or coactivator-associated arginine methyltransferase 1) [30] in cells. H3R17 methylation by PRMT4 activates gene expression, and the repressive function of PADI4 on target genes has been linked to the negative influence on H3R17 methylation and its association with HDAC2 [35] . However, citrullination of H3R8 by PADI4 can result in activation due to inhibition of HP1 binding [36] . Recently, citrullination of H4R3 by PADI4 has been linked to the p53 pathway [37] . A genome-wide analysis of PADI4 activity revealed that PADI4 can associate with active genes and act as an activator of gene expression by citrullination of transcription factors [38] . These results argue for a context-specific repressive or activating transcriptional cofactor activity of PADI4. PADI4 expression has been detected in human CD34+ stem cell/progenitor cells [39] , and PADI4 plays a role in regulation of hematopoietic progenitor proliferation [40] . Recently, it was shown that PADI4 is part of a transcriptional network, which regulates pluripotency [41] . In cancer, high PADI4 expression was connected to tumor growth and the PADI4 inhibitor Cl-amidine reduces growth of a subset of cell lines [42] . In this study we identified PADI4 as an interaction partner of Tal1 by affinity purification and subsequent stable isotope labelling by amino acids in cell culture (SILAC)-based mass spectrometric identification of co-purified proteins [43] . For this approach, we used the high-affinity biotin-tag birA-ligase system [11] , [23] , [44] . By knockdown of PADI4 and Tal1 in the erythroleukemia cell line HEL, we identified co-regulated genes and direct Tal1/PADI4 target genes. We found that Tal1 and PADI4 are bound to the promoters of IL6ST (interleukin 6 signal transducer, gp130), which mediates IL6 signalling, and CTCF (CCCTC-binding factor), a central transcriptional regulator [45] , [46] , [47] , [48] . In particular, we demonstrate that PADI4 acts as a coactivator of Tal1 by counteracting the repressive H3R2me2a mark at the IL6ST promoter. This novel function of PADI4 sheds light on the mechanisms of gene regulation by the central hematopoietic transcription factor Tal1. PADI4 is a novel Tal1 interaction partner For identification of Tal1 interaction partners, we combined affinity purification using the birA-biotin tag system with quantitative mass spectrometric analysis using SILAC [43] . Erythroleukemia cells harbouring the birA-ligase together with a bir-tagged Tal1 (bir-Tal1) were grown in heavy SILAC medium (H) [10] . In vivo biotinylated bir-Tal1 protein was affinity purified using streptavidine beads and mixed in equimolar amounts with a control sample from birA-ligase cells, which were grown in light SILAC medium (L). Purified Tal1 and copurified proteins were separated by one-dimensional-polyacrylamide gel electrophoresis (PAGE) and proteins were identified by mass spectrometry. The relative abundance of proteins in the bir-Tal1 sample compared with the birA-ligase only cells was determined by calculating the ratio between peak intensities of identified peptides from the heavy (H, bir-Tal1) versus the light (L, birA-ligase) sample. An H/L ratio of >5 was considered as a highly significant enrichment in the bir-Tal1 sample. A detailed scheme of the experimental procedure is given ( Supplementary Fig. 1 ). Besides Tal1 itself, we identified known members of Tal1 complexes such as MTGR1, MTG16 (ETO2), LDB1, LMO2 and the basic helix-loop-helix transcription factors HEB, E2-2 and E47 (E2A) ( Fig. 1a ). Furthermore, the single-stranded DNA-binding proteins 3 and 4 (SSBP3 and SSBP4) and the nucleosome assembly protein 1-like-4 were identified. 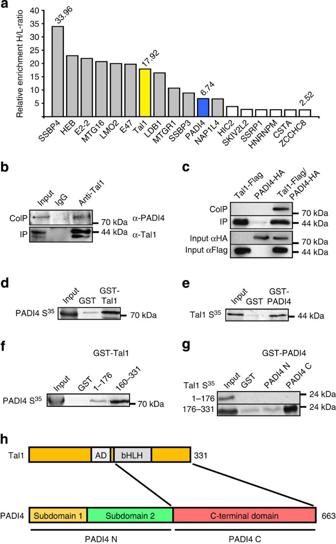Figure 1: PADI4 is a novel Tal1 interaction partner. (a) Identification of members of the Tal1 interactome by affinity purification and SILAC-based MS analysis. Proteins that showed an enrichment of heavy (H)- to light (L)-labelled peptides above 5 (ratio H/L >5) were identified as components of the Tal1 interactome in the SILAC-based MS analysis and are marked in grey, yellow (Tal1) and blue (PADI4). Further not significant enriched proteins with an H/L ratio of fivefold to 2.5-fold are shown. Detailed information including total number of all identified and quantified proteins is provided inSupplementary Data 1. (b) Endogenous Tal1 interacts with endogenous PADI4 in HEL cells. Immunoprecipitation (IP) was performed using an anti-Tal1 antibody, coimmunoprecipitated (CoIP) PADI4 was detected with an anti-PADI4 antibody. (c) Tal1 interacts with PADI4 in a CoIP performed with lysates of transfected HEK293 cells. IP was performed with anti-Flag M2 beads, which pulls out Flag-Tal1. Coimmunoprecitated HA-tagged PADI4 was detected with an anti-HA antibody. (d,e)In vitrotranslated PADI4 interacts with GST-Tal1 andin vitrotranslated Tal1 interacts with GST-PADI4 in a GST-pulldown. (f) Interaction of the C terminus of Tal1 with PADI4 in GST-pulldown. (g) Interaction of the C terminus of PADI4 with the C terminus of Tal1 in GST-pulldown. (h) Schematic representation of the interaction between Tal1 and PADI4. The approximate position of proteins is given. Figure 1a shows significantly enriched proteins (ratio H/L>5) and proteins with an H/L ratio between 2.5 and 5. An extended list of identified and quantified proteins is given in ( Supplementary Table 1 ) as well as a complete list is provided in the ( Supplementary Data 1 ). Figure 1: PADI4 is a novel Tal1 interaction partner. ( a ) Identification of members of the Tal1 interactome by affinity purification and SILAC-based MS analysis. Proteins that showed an enrichment of heavy (H)- to light (L)-labelled peptides above 5 (ratio H/L >5) were identified as components of the Tal1 interactome in the SILAC-based MS analysis and are marked in grey, yellow (Tal1) and blue (PADI4). Further not significant enriched proteins with an H/L ratio of fivefold to 2.5-fold are shown. Detailed information including total number of all identified and quantified proteins is provided in Supplementary Data 1 . ( b ) Endogenous Tal1 interacts with endogenous PADI4 in HEL cells. Immunoprecipitation (IP) was performed using an anti-Tal1 antibody, coimmunoprecipitated (CoIP) PADI4 was detected with an anti-PADI4 antibody. ( c ) Tal1 interacts with PADI4 in a CoIP performed with lysates of transfected HEK293 cells. IP was performed with anti-Flag M2 beads, which pulls out Flag-Tal1. Coimmunoprecitated HA-tagged PADI4 was detected with an anti-HA antibody. ( d , e ) In vitro translated PADI4 interacts with GST-Tal1 and in vitro translated Tal1 interacts with GST-PADI4 in a GST-pulldown. ( f ) Interaction of the C terminus of Tal1 with PADI4 in GST-pulldown. ( g ) Interaction of the C terminus of PADI4 with the C terminus of Tal1 in GST-pulldown. ( h ) Schematic representation of the interaction between Tal1 and PADI4. The approximate position of proteins is given. Full size image Interestingly, PADI4 was identified as a potential Tal1-associated protein ( Fig. 1a ; Supplementary Fig. 2 ). PADI4 is an epigenetic enzyme, which converts arginine residues at histone tails to citrulline [29] . Because we are especially interested in epigenetic mechanisms connected to Tal1, we further analysed the Tal1/PADI4 association. We could show the interaction of Tal1 with PADI4 at the endogenous level from the erythroleukemia cell line HEL ( Fig. 1b ). We verified the interaction of Tal1 with PADI4 by coimmunoprecipitation (CoIP) in transiently transfected HEK293 cells ( Fig. 1c ). Interaction between the proteins was also shown in a glutathione S -transferase (GST)-pulldown with in vitro -translated PADI4 and in Escherichia coli produced GST-Tal1, and vice versa ( Fig. 1d,e ). The main interaction domain of Tal1 with PADI4 is located within the C terminus of the protein. The C-terminal GST-Tal1 construct of amino acids 160–331 interacted stronger with full-length PADI4 than the N-terminal GST-Tal1 of amino acids 1–176 ( Fig. 1f ). The interaction domain on the PADI4 side involves the C-terminus of PADI4 [49] , which displayed a robust interaction with the C terminus of Tal1 ( Fig. 1g ). Taken together, we identified PADI4 as a novel interaction partner of Tal1 and the C-terminal parts of the proteins mediate this interaction ( Fig. 1h ). PADI4 and Tal1 coinfluence gene expression To functionally analyse Tal1 interaction with PADI4, we knocked down PADI4 and Tal1 by short hairpin RNA (shRNA) in HEL cells. Knockdown was confirmed by a reduction of Tal1 and PADI4 at the messenger RNA (mRNA) and protein levels ( Fig. 2a,b ; Supplementary Fig. 3 ). Subsequently, we performed microarray gene expression analysis. Knockdown of Tal1 altered expression of 1,203 genes and knockdown of PADI4 changed expression of 702 genes ( Fig. 2c ). When we merged the gene lists of Tal1- and PADI4-influenced genes, we found that the expression of 414 genes was differentially regulated in both data sets ( Fig. 2d ). 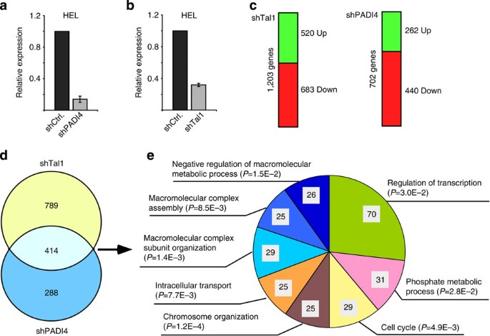Figure 2: Gene expression analysis upon Tal1 and PADI4 knockdown. (a) HEL cells were transduced with shRNAs against PADI4 (shPADI4) and the knockdown evaluated by quantitative real-time PCR. Error bars represent the s.d. of at least four determinations from two independent transductions. (b) HEL cells were transduced with shRNAs against Tal1 (shTal1) and the knockdown evaluated by quantitative real-time PCR. Error bars represent the s.d. of at least four determinations from two independent transductions. (c) Gene expression array analysis was performed with shTal1 and shPADI4 cells. Knockdown of Tal1 altered expression of 1,203 genes and knockdown of PADI4 altered expression of 702 genes. (d) Comparison of Tal1- and PADI4-influenced genes. Genes (414) are changed in both data sets. (e) Gene ontology analysis of the 414 genes changed upon Tal1 and PADI4 knockdown. The pie chart gives the enriched GO-terms (GO-term-BP) with the highest numbers of included genes. Analysis was performed using DAVID using standard settings.P-values are given. Figure 2: Gene expression analysis upon Tal1 and PADI4 knockdown. ( a ) HEL cells were transduced with shRNAs against PADI4 (shPADI4) and the knockdown evaluated by quantitative real-time PCR. Error bars represent the s.d. of at least four determinations from two independent transductions. ( b ) HEL cells were transduced with shRNAs against Tal1 (shTal1) and the knockdown evaluated by quantitative real-time PCR. Error bars represent the s.d. of at least four determinations from two independent transductions. ( c ) Gene expression array analysis was performed with shTal1 and shPADI4 cells. Knockdown of Tal1 altered expression of 1,203 genes and knockdown of PADI4 altered expression of 702 genes. ( d ) Comparison of Tal1- and PADI4-influenced genes. Genes (414) are changed in both data sets. ( e ) Gene ontology analysis of the 414 genes changed upon Tal1 and PADI4 knockdown. The pie chart gives the enriched GO-terms (GO-term-BP) with the highest numbers of included genes. Analysis was performed using DAVID using standard settings. P -values are given. Full size image Gene ontology analysis of the 414 common genes using DAVID [50] revealed that the largest number of these is involved in regulation of transcription ( Fig. 2e ). Within the regulated genes with the most strongly enriched gene ontology (GO)-term categories were genes involved in leukocyte differentiation, chromosome organization and hemopoiesis ( Table 1 ). Of 414 common genes, 162 genes were upregulated and 248 were downregulated upon Tal1 and PADI4 knockdown. The large number of co-regulated genes is consistent with an intricate relationship of Tal1 and PADI4 in gene regulation. When we compared the list of 414 Tal1- and PADI4-influenced genes from HEL erythroleukemia cells with recently identified direct Tal1 target genes in the murine hematopoietic cell line HPC-7 [21] , we found that 162 genes were already described as direct Tal1 target genes in HPC-7 cells. Table 1 GO-terms with the most significant enrichment. Full size table We reanalysed Tal1/PADI4-regulated genes, which are involved in leukocyte differentiation and hematopoiesis (compare Table 1 ) by quantitative reverse transcriptase-PCR ( Supplementary Fig. 4 ). CTCF , FGFR1OP2 and TNF were upregulated upon Tal1 or PADI4 knockdown ( Fig. 3a–c ); IL6ST , CEBP ε and VEGFA were downregulated upon Tal1 or PADI4 knockdown ( Fig. 3d–f ). 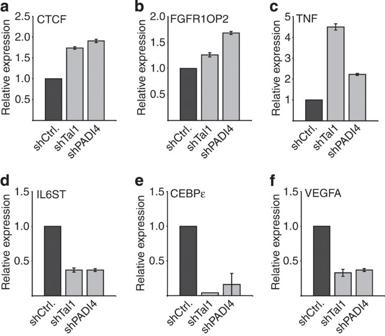Figure 3: Verification of gene expression changes upon Tal1 and PADI4 knockdown. (a–f) A subset of genes from the array analysis was reanalysed by quantitative real-time PCR. Error bars represent the s.d. from at least four determinations and two independent knockdowns. Figure 3: Verification of gene expression changes upon Tal1 and PADI4 knockdown. ( a – f ) A subset of genes from the array analysis was reanalysed by quantitative real-time PCR. Error bars represent the s.d. from at least four determinations and two independent knockdowns. Full size image Subsequently, we performed chromatin immunoprecipitation (ChIP) using specific antibodies against Tal1 or PADI4 to determine whether identified genes are direct target genes of Tal1 or PADI4. Guided by published ChIP-seq data, we designed primer pairs covering E-boxes at the promoters of identified genes and detected Tal1 and PADI4 binding to the promoter regions of IL6ST and CTCF by ChIP ( Fig. 4 ; Supplementary Fig. 5 ). 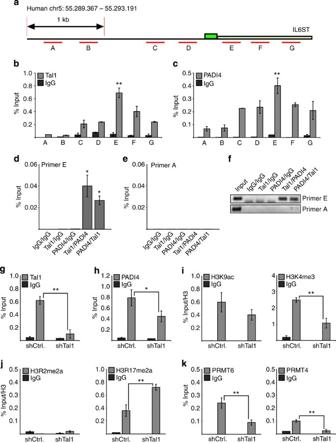Figure 4:Analysis of Tal1 and PADI4 binding to theIL6ST5′-region and influence of Tal1. (a) Schematic representation of the analysedIL6STgenomic locus including the 5′-region. The genomic position is given and the position of primer pairs used for ChIP analysis is indicated. The first non-coding exon is marked in dark green and the first intron in light green. (b) Mapping of Tal1 binding to theIL6ST5′-region. Upon ChIP with an anti-Tal1 antibody qPCR with primers at different positions of the IL6ST 5′-region was performed. (c) ChIP shows binding of PADI4 to theIL6ST5′-region. Upon ChIP with an anti-PADI4 antibody qPCR with primers at different positions of the IL6ST 5′-region was performed. TheP-value gives the statistical significant difference between the values gathered with primer E compared with primer A. (d–f) Analysis of concomitant Tal1 and PADI4 binding to theIL6ST5′-region by ChIP-ReChIP. (d) Concomitant Tal1 and PADI4 binding is detected at a region close to the first exon ofIL6ST(primer E). (e) No Tal1/PADI4 is detected with an upstream primer (primer A). (f) Analysis of the ChIP-ReChIP qPCR products by gel electrophoresis at the end point of the qPCR reaction confirms qPCR results. Antibody combinations and primer pairs are given. TheP-value (*P<0.05) gives the statistical significant enrichment of the ChIP-ReChIP compared with the IgG controls according to Student’st-test. (g) ChIP demonstrates decreased Tal1 binding to theIL6STpromoter upon Tal1 knockdown. (h) ChIP shows decreased PADI4 binding to theIL6STpromoter upon Tal1 knockdown. (i) The histone modification marks H3K9ac and H3K4me3 are decreased upon Tal1 knockdown at the IL6ST promoter. (j) The histone modification H3R2me2a remains at a low level upon Tal1 knockdown and H3R17me2a is increased at the IL6ST promoter. (k) PRMT6 and PRMT4 binding are decreased upon Tal1 knockdown at the IL6ST promoter. Values are shown as percent enrichment compared with the input. Error bars represent the s.d. from at least four determinations. TheP-values were calculated using thet-test, *P<0.05, **P<0.01. Figure 4a indicates the genomic position of the analysed promoter region of IL6ST and the location of primers for subsequent ChIP analysis. Using primer pairs at different locations at the IL6ST promoter for ChIP-qPCR analysis, we mapped Tal1 binding to the IL6ST promoter to the proximity of the first non-coding exon of IL6ST ( Fig. 4b ). Similarly, PADI4 binding was localized to the same region of the IL6ST promoter ( Fig. 4c ). To determine whether Tal1 and PADI4 concomitantly bind to the IL6ST promoter, we performed ChIP-ReChIP analysis and could detect Tal1 and PADI4 together close to the transcriptional start site but not at a downstream region, which served as a negative control ( Fig. 4d–f ). A similar analysis was performed for CTCF ( Supplementary Fig. 5 ). Figure 4: Analysis of Tal1 and PADI4 binding to the IL6ST 5′-region and influence of Tal1. ( a ) Schematic representation of the analysed IL6ST genomic locus including the 5′-region. The genomic position is given and the position of primer pairs used for ChIP analysis is indicated. The first non-coding exon is marked in dark green and the first intron in light green. ( b ) Mapping of Tal1 binding to the IL6ST 5′-region. Upon ChIP with an anti-Tal1 antibody qPCR with primers at different positions of the IL6ST 5′-region was performed. ( c ) ChIP shows binding of PADI4 to the IL6ST 5′-region. Upon ChIP with an anti-PADI4 antibody qPCR with primers at different positions of the IL6ST 5′-region was performed. The P -value gives the statistical significant difference between the values gathered with primer E compared with primer A. ( d – f ) Analysis of concomitant Tal1 and PADI4 binding to the IL6ST 5′-region by ChIP-ReChIP. ( d ) Concomitant Tal1 and PADI4 binding is detected at a region close to the first exon of IL6ST (primer E). ( e ) No Tal1/PADI4 is detected with an upstream primer (primer A). ( f ) Analysis of the ChIP-ReChIP qPCR products by gel electrophoresis at the end point of the qPCR reaction confirms qPCR results. Antibody combinations and primer pairs are given. The P -value (* P <0.05) gives the statistical significant enrichment of the ChIP-ReChIP compared with the IgG controls according to Student’s t -test. ( g ) ChIP demonstrates decreased Tal1 binding to the IL6ST promoter upon Tal1 knockdown. ( h ) ChIP shows decreased PADI4 binding to the IL6ST promoter upon Tal1 knockdown. ( i ) The histone modification marks H3K9ac and H3K4me3 are decreased upon Tal1 knockdown at the IL6ST promoter. ( j ) The histone modification H3R2me2a remains at a low level upon Tal1 knockdown and H3R17me2a is increased at the IL6ST promoter. ( k ) PRMT6 and PRMT4 binding are decreased upon Tal1 knockdown at the IL6ST promoter. Values are shown as percent enrichment compared with the input. Error bars represent the s.d. from at least four determinations. The P -values were calculated using the t -test, * P <0.05, ** P <0.01. Full size image To evaluate the contribution of Tal1 on transcription, we performed ChIP experiments upon knockdown of Tal1. Knockdown of Tal1 resulted in diminished Tal1 occupancy on the IL6ST promoter ( Fig. 4g ). PADI4 binding is decreased upon knockdown of Tal1, which indicates that Tal1 takes part in PADI4 recruitment ( Fig. 4h ). Furthermore, knockdown resulted in reduced presence of the active histone marks H3K9ac and H3K4me3 ( Fig. 4i ), which is in line with the downregulation of IL6ST expression upon loss of Tal1 (compare Fig. 3 ). The repressive H3R2me2a mark is unchanged upon Tal1 knockdown and the active H3R17me2a mark is increased ( Fig. 4j ). Moreover, we observed that PRMT6 and PRMT4 binding is slightly reduced upon Tal1 knockdown ( Fig. 4k ). Taken together, we confirmed IL6ST and CTCF as direct Tal1/PADI4 target genes. CTCF is a central regulator of gene expression and plays a role at the megakaryocytic/erythrocytic branching point [45] , [46] , [47] , [48] . IL6ST (gp130) is an important transducer of cytokine signalling, which plays a central role in hematopoiesis and is a target molecule for cancer therapy [51] , [52] , [53] , [54] . PADI4 influences histone arginine methylation PADI4 can modify histone arginines by citrullination and thus counteract arginine methylation by PRMTs. Because CTCF and IL6ST expression are differentially effected upon Tal1 and PADI4 knockdown, we performed a site-by-site comparison of the histone modification status of the CTCF and IL6ST promoters after PADI4 knockdown. As expected, upon knockdown of PADI4 by shRNA the amount of PADI4 on the promoters of CTCF and IL6ST was strongly reduced ( Fig. 5a ), while Tal1 occupancy was not changed significantly ( Fig. 5b ). PADI4 is able to counteract the active H3R17me2a mark, which is mediated by PRMT4. H3R17me2a increased to a robust level on the CTCF promoter and on the IL6ST promoter already some H3R17me2a was detected, which was further increased upon PADI4 knockdown ( Fig. 5c ). Concomitantly, we detected an increase of PRMT4 occupancy on the CTCF and IL6ST promoters ( Fig. 5d ). 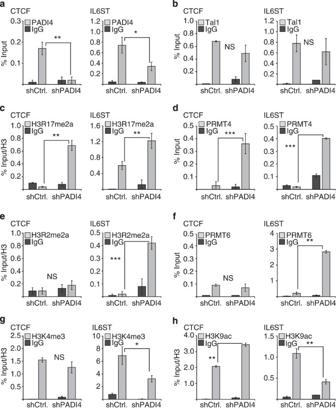Figure 5:Epigenetic changes upon PADI4 knockdown at theCTCFandIL6STpromoter. (a) ChIP demonstrates decreased PADI4 occupancy of theCTCFandIL6STpromoters upon PADI4 knockdown. (b) ChIP shows no changes in Tal1 binding to theCTCFandIL6STpromoters upon PADI4 knockdown. (c) The PRMT4-mediated H3R17me2a mark is increased upon PADI4 knockdown at theCTCFandIL6STpromoters. (d) PRMT4 binding is increased at theCTCFandIL6STpromoters upon PADI4 knockdown. (e) H3R2me2a is increased upon PADI4 knockdown at theIL6STpromoter, but not at theCTCFpromoter. (f) PRMT6 binding is increased at theIL6STpromoter upon PADI4 knockdown. (g) The H3K4me3 histone mark is significantly decreased at theIL6STpromoter. (h) The positive histone mark H3K9ac decreases upon PADI4 knockdown at theIL6STpromoter. Values are shown as percent enrichment compared with the input. Error bars represent the s.d. from at least four determinations. TheP-values were calculated using thet-test, *P<0.05, **P<0.01, ***P<0.001. NS, not significant. Figure 5: Epigenetic changes upon PADI4 knockdown at the CTCF and IL6ST promoter. ( a ) ChIP demonstrates decreased PADI4 occupancy of the CTCF and IL6ST promoters upon PADI4 knockdown. ( b ) ChIP shows no changes in Tal1 binding to the CTCF and IL6ST promoters upon PADI4 knockdown. ( c ) The PRMT4-mediated H3R17me2a mark is increased upon PADI4 knockdown at the CTCF and IL6ST promoters. ( d ) PRMT4 binding is increased at the CTCF and IL6ST promoters upon PADI4 knockdown. ( e ) H3R2me2a is increased upon PADI4 knockdown at the IL6ST promoter, but not at the CTCF promoter. ( f ) PRMT6 binding is increased at the IL6ST promoter upon PADI4 knockdown. ( g ) The H3K4me3 histone mark is significantly decreased at the IL6ST promoter. ( h ) The positive histone mark H3K9ac decreases upon PADI4 knockdown at the IL6ST promoter. Values are shown as percent enrichment compared with the input. Error bars represent the s.d. from at least four determinations. The P -values were calculated using the t -test, * P <0.05, ** P <0.01, *** P <0.001. NS, not significant. Full size image Interestingly, upon PADI4 knockdown we detected the appearance of the repressive H3R2me2a mark at the IL6ST promoter, the opposite of what we observed at the CTCF promoter ( Fig. 5e ). At the same time, we found an increased occupancy of PRMT6 at the IL6ST promoter, but not at the CTCF promoter ( Fig. 5f ). PRMT6-mediated H3R2me2a acts in an inhibitory fashion on the H3K4me3 mark. In agreement with this notion, we found the activating H3K4me3 mark unchanged in the case of CTCF and decreased in the case of IL6ST ( Fig. 5g ). In addition, we analysed the H4R3me2a status, which was recently connected to PADI4 activity [37] . H4R3me2a was increased on the CTCF and IL6ST promoter upon PADI4 knockdown ( Supplementary Fig. 6 ). The activating histone mark H3K9ac increased at the CTCF promoter and decreased at the IL6ST promoter ( Fig. 5h ), which is in agreement with observed expression changes (compare Fig. 3 ; Supplementary Fig. 3 for changes of IL6ST surface expression). Altogether, we found that PADI4 acts repressively on CTCF expression by keeping the activating H3R17me2a histone mark at a low level. In contrast, the main effect of PADI4 on the IL6ST promoter was suppression of the repressive H3R2me2a mark, which counteracts H3K4me3. By this mechanism PADI4 acts as an activator of IL6ST expression. These data show that PADI4 influences the epigenetic status of Tal1-target regulatory elements by changing arginine methylation patterns at distinct histone arginines. Pharmacological inhibition of PADI4 Our data show that PADI4 negatively influences expression of Tal1 target genes such as CTCF and promotes transcriptional activation of others, such as IL6ST . IL6ST (gp130) is an important transducer of cytokine signalling, for example, triggered by interleukin (IL)-6. Furthermore, IL6ST has a role in self-renewal of HSCs and hematopoietic differentiation [51] , [53] . In addition, IL6ST signalling contributes to growth control and is thus regarded as a promising target for cancer therapy [54] , [55] . The small-molecule Cl-amidine inhibits PADI4 activity [56] . Treatment of HEL cells with Cl-amidine changed a subset of leukocyte or hematopoiesis-associated genes, which were altered upon Tal1 or PADI4 knockdown ( Supplementary Fig. 4 ). Notably, pharmacological inhibition of PADI4 by Cl-amidine decreased IL6ST expression in HEL cells ( Fig. 6a ). Treatment with Cl-amidine did not immediately influence growth of HEL cells, but on day 9 of treatment a significant decrease in cell numbers compared with the mock control was observed ( Supplementary Fig. 7 ). Other cell lines also displayed sensitivity to Cl-amidine ( Supplementary Fig. 7 ). Upon Cl-amidine treatment, the amount of Tal1 and PADI4 on the IL6ST promoter was slightly reduced ( Fig. 6b,c ). In agreement with our data gathered upon PADI4 knockdown, we detected a strong increase in H3R2me2a upon inhibitor treatment ( Fig. 6d , compare Figure 5e ). Consistent with the notion that H3R2me2a inhibits the H3K4me3 mark, we also detected a significant decrease in H3K4me3 on the IL6ST promoter ( Fig. 6e ). H3R17me2a did not change upon inhibitor treatment ( Fig. 6f ). In contrast, at the CTCF promoter H3R17me2a was increased and H3R2me2a remained unchanged upon Cl-amidine treatment ( Fig. 6g,h ). 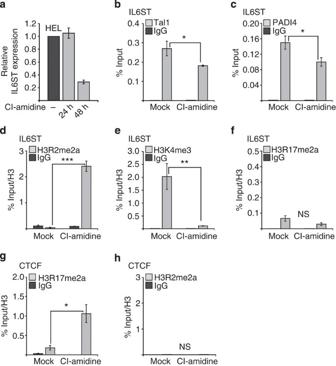Figure 6:The PADI4 inhibitor Cl-amidine influencesIL6STgene expression and epigenetic marking. (a)IL6STexpression is decreased upon treatment of HEL cells with Cl-amidine (200 μM) for 48 h. (b) Tal1 occupancy of theIL6STpromoter upon Cl-amidine treatment of HEL cells measured by ChIP. (c) PADI4 occupancy of theIL6STpromoter upon Cl-amidine treatment of HEL cells measured by ChIP. (d) The negative histone mark H3R2me2a is increased at theIL6STpromoter upon Cl-amidine treatment of HEL cells measured by ChIP. (e) H3K4me3 is decreased at theIL6STpromoter upon Cl-amidine treatment in HEL cells. (f) H3R17me2a at theIL6STpromoter is unaffected by Cl-amidine treatment. (g,h) In contrast to theIL6STpromoter, at theCTCFpromoter H3R17me2a was increased and H3R2me2a remained unchanged upon Cl-amidine treatment. Values are shown as percent enrichment compared with the input. Error bars represent the s.d. of at least four determinations. TheP-values were calculated using thet-test, *P<0.05, **P<0.01, ***P<0.001. NS, not significant. Figure 6: The PADI4 inhibitor Cl-amidine influences IL6ST gene expression and epigenetic marking. ( a ) IL6ST expression is decreased upon treatment of HEL cells with Cl-amidine (200 μM) for 48 h. ( b ) Tal1 occupancy of the IL6ST promoter upon Cl-amidine treatment of HEL cells measured by ChIP. ( c ) PADI4 occupancy of the IL6ST promoter upon Cl-amidine treatment of HEL cells measured by ChIP. ( d ) The negative histone mark H3R2me2a is increased at the IL6ST promoter upon Cl-amidine treatment of HEL cells measured by ChIP. ( e ) H3K4me3 is decreased at the IL6ST promoter upon Cl-amidine treatment in HEL cells. ( f ) H3R17me2a at the IL6ST promoter is unaffected by Cl-amidine treatment. ( g , h ) In contrast to the IL6ST promoter, at the CTCF promoter H3R17me2a was increased and H3R2me2a remained unchanged upon Cl-amidine treatment. Values are shown as percent enrichment compared with the input. Error bars represent the s.d. of at least four determinations. The P -values were calculated using the t -test, * P <0.05, ** P <0.01, *** P <0.001. NS, not significant. Full size image To evaluate the influence of PADI4 on IL6ST expression in primary cells, we examined PADI4 and IL6ST expression during differentiation of human CD34+ progenitor cells. We observed upregulation of IL6ST expression during erythroid and monocytic differentiation ( Fig. 7a ). IL6ST mRNA levels remained unchanged upon megakaryocytic differentiation compared with non-induced cells ( Fig. 7a ). Tal1 binding to the IL6ST promoter remained similar during erythroid or megakaryocytic differentiation and was slightly decreased upon monocytic differentiation ( Fig. 7b ). Concomitantly with upregulation of IL6ST , we detected increased binding of PADI4 to the IL6ST promoter upon erythroid and monocytic differentiation ( Fig. 7c ). During megakaryocytic differentiation PADI4 binding was decreased ( Fig. 7c ) and H3R2me2a increased ( Fig. 7d ). During erythroid and monocytic differentiation H3R2me2a was slightly decreased. These data are in agreement with our results gathered in HEL cells, which implicate that PADI4 acts in an activating manner on IL6ST expression (compare Fig. 5 ). Subsequently, we examined whether PADI4 influences hematopoietic differentiation of hCD34+ cells in a colony-formation assay. When we overexpressed PADI4, we observed fewer monocytic colonies, whereas an enzymatically inactive mutant did not show this effect ( Fig. 7e ). Inversely, knockdown of PADI4 increased the number of monocytic colonies ( Fig. 7f ). 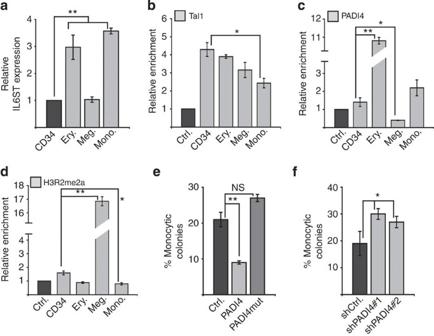Figure 7:IL6STexpression changesduring differentiation of hCD34+ cells that correlate with PADI4 recruitment and epigenetic alterations. (a)IL6STexpression is increased upon erythroid and monocytic differentiation of primary human CD34+ cells and remains unchanged upon megakaryocytic differentiation. (b) Tal1 binding to theIL6STpromoter is unchanged upon erythroid and megakaryocytic differentiation. (c) PADI4 binding to theIL6STpromoter increased upon erythroid and monocytic differentiation and decreased upon megakaryocytic differentiation. (d) The repressive H3R2me2a mark is strongly upregulated upon megakaryocytic differentiation and decreased upon erythroid and monocytic differentiation. ChIP assays were performed with at least two independent preparations and measured in duplicates. Values are shown normalized to the input and as relative enrichment over background. (e) Influence of PADI4 on hematopoietic colony formation. Overexpression of PADI4 reduces the number of monocytic colonies in a CFU-C assay. An enzymatic inactive PADI4 mutant does not inhibit monocytic differentiation. (f) Knock down of PADI4 increases the number of monocytic colonies in a colony-formation unit-C assay. hCD34+ cells were expanded for 4 days, transduced and sorted according to their green fluorescent protein signal. Subsequently, the transduced cells were seeded in methocult. Colonies were evaluated 2 weeks after seeding. Error bars represent the s.d. of three determinations. TheP-values were calculated using thet-test, *P<0.05, **P<0.01. NS, not significant. Figure 7: IL6ST expression changes during differentiation of hCD34+ cells that correlate with PADI4 recruitment and epigenetic alterations. ( a ) IL6ST expression is increased upon erythroid and monocytic differentiation of primary human CD34+ cells and remains unchanged upon megakaryocytic differentiation. ( b ) Tal1 binding to the IL6ST promoter is unchanged upon erythroid and megakaryocytic differentiation. ( c ) PADI4 binding to the IL6ST promoter increased upon erythroid and monocytic differentiation and decreased upon megakaryocytic differentiation. ( d ) The repressive H3R2me2a mark is strongly upregulated upon megakaryocytic differentiation and decreased upon erythroid and monocytic differentiation. ChIP assays were performed with at least two independent preparations and measured in duplicates. Values are shown normalized to the input and as relative enrichment over background. ( e ) Influence of PADI4 on hematopoietic colony formation. Overexpression of PADI4 reduces the number of monocytic colonies in a CFU-C assay. An enzymatic inactive PADI4 mutant does not inhibit monocytic differentiation. ( f ) Knock down of PADI4 increases the number of monocytic colonies in a colony-formation unit-C assay. hCD34+ cells were expanded for 4 days, transduced and sorted according to their green fluorescent protein signal. Subsequently, the transduced cells were seeded in methocult. Colonies were evaluated 2 weeks after seeding. Error bars represent the s.d. of three determinations. The P -values were calculated using the t -test, * P <0.05, ** P <0.01. NS, not significant. Full size image Taken together, PADI4 can act as an activator of Tal1-target gene expression, such as IL6ST , by counteracting H3R2me2a methylation triggered by PRMT6 ( Fig. 8a ). In contrast, at distinct target genes PADI4 is a repressor of gene expression ( Fig. 8b ). 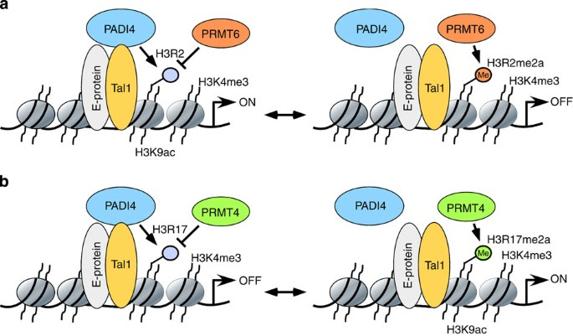Figure 8:Model of PADI4 activity with Tal1 on regulatory elements of genes, such asIL6STandCTCF. (a) PADI4 as an activator. Tal1 recruits PADI4, which inhibits H3R2me2a by PRMT6. As a consequence H3K4me3 remains at a high level and the gene is transcribed. Upon loss of PADI4 binding H3R2me2a is triggered by PRMT6. Subsequently, the H3K4me3 level is decreased and expression downregulated. (b) PADI4 as a repressor. Tal1 recruits PADI4, which inhibits H3R17me2a by PRMT4 and contributes to low expression of the gene. Upon loss of PADI4 binding H3R17me2a is triggered by PRMT4. Subsequently, the H3K4me3 level increases and expression is upregulated. Figure 8: Model of PADI4 activity with Tal1 on regulatory elements of genes, such as IL6ST and CTCF. ( a ) PADI4 as an activator. Tal1 recruits PADI4, which inhibits H3R2me2a by PRMT6. As a consequence H3K4me3 remains at a high level and the gene is transcribed. Upon loss of PADI4 binding H3R2me2a is triggered by PRMT6. Subsequently, the H3K4me3 level is decreased and expression downregulated. ( b ) PADI4 as a repressor. Tal1 recruits PADI4, which inhibits H3R17me2a by PRMT4 and contributes to low expression of the gene. Upon loss of PADI4 binding H3R17me2a is triggered by PRMT4. Subsequently, the H3K4me3 level increases and expression is upregulated. Full size image During hematopoietic differentiation chromatin is extensively reorganized and epigenetic marks are adjusted. This contributes to epigenetic refinement of gene expression programs during differentiation. Transcription factors play a decisive role in the assembly of gene and cell-specific transcriptional complexes, and their deregulation can result in uncontrolled cell growth and subsequently cancer. Consequently, small-molecule inhibitors of epigenetic cofactors such as histone deacetylase inhibitors are highly desired. The transcription factor Tal1 is a critical regulator of hematopoietic gene expression and can act as an oncogene if aberrantly expressed. In this work, we have identified PADI4 as a novel interaction partner of Tal1 and we found that a large number of genes are co-regulated by Tal1 and PADI4. Strikingly, we identified genes that are concomitantly downregulated by Tal1 or PADI4 knockdown as well as concurrently upregulated genes. This observation strengthens the notion of a close functional connection between Tal1 and PADI4, and also demonstrates the existence of a repressive and an activating mode of cooperation between Tal1 and PADI4. PADI4 is able to citrullinate monomethylated arginine residues at histones and thus counteracts the activity of PRMTs [30] , [31] . As was previously shown, H3R17 deimination by PADI4 counteracts H3R17 methylation by PRMT4 [57] . This block of H3R17 methylation has a repressive effect, as a consequence PADI4 acts as a corepressor of gene expression on these genes. This is in line with our observation that knockdown of PADI4 increases PRMT4 recruitment and H3R17 methylation on the CTCF promoter and augments CTCF gene expression. Thus on the CTCF promoter PADI4 exerts inhibitory effects on expression by counteracting H3R17me2a. Because some degree of CTCF expression was detectable in the presence of PADI4, a possible scenario is dynamic competition of PADI4 and PRMT4 for access to H3R17. Unexpectedly, upon PADI4 knockdown we observed a strong increase of H3R2me2a at the IL6ST promoter. This increase of the repressive H3R2me2a histone mark [58] , [59] , [60] goes hand-in-hand with downregulation of IL6ST expression. H3R2me2a mediated by PRMT6 is able to inhibit the prominent H3K4me3 mark [58] , [59] , [60] , [61] , [62] . In agreement with this notion, we detected decreased H3K4me3 methylation concomitant with the upregulation of H3R2me2a upon PADI4 knockdown. This is the first report of an involvement of PADI4 in repression of the H3R2me2a mark and an indirect support of the H3K4me3 mark by PADI4. Interestingly, we could also detect an increase of the repressive H3R2me2a mark, a decrease of H3K4me3 and a concomitant downregulation of IL6ST expression, when we pharmacologically inhibited PADI4 with the small-molecule compound Cl-amidine. Notably, the slight increase of H3R17me2a upon PADI4 knockdown at the IL6ST promoter was not detectable upon Cl-amidine treatment. This could indicate that the presence of PADI4 protein also influences complex formation structurally. Furthermore, we found that during differentiation of primary human CD34+ progenitor cells IL6ST expression is correlated with PADI4 occupancy of the IL6ST promoter. Low PADI4 occupancy during megakaryocytic differentiation is related to high levels of H3R2me2a. This result demonstrates that increased PADI4 binding can be associated with gene activation during differentiation. Our observation that PADI4 influences monocytic differentiation in a colony-formation assay shows that the function of PADI4 might be critical for hematopoietic differentiation. The observation that a number of genes important for leukocyte differentiation such as CEBPε are changed upon Tal1 and PADI4 knockdown, could offer an explanation for the influence of PADI4 on differentiation. Interestingly, it was recently demonstrated that PADI4 regulates c-myc expression in conjunction with the transcription factor LEF1 and in this manner influences multipotent hematopoietic progenitor proliferation [40] . For the detailed analysis of PADI4 function in distinct hematopoietic lineages, cell-type-specific PADI4 knockout in the mouse model will be required. Taken together, PADI4 can target different histone arginines [30] , [31] and our data support the notion of a function of PADI4 as a general opponent of PRMTs. Thus, PADI4 might act as a repressor if activating arginine methylation is inhibited, or an activator if the balance of PADI4 activity is shifted towards suppression of repressive arginine methylation. In this regard, our data show that PADI4 contributes to epigenetic fine-tuning of Tal1 target gene expression in hematopoiesis. A further advance in this field of study would be the identification of an enzyme that reverses citrullination by PADI4 and would facilitate renewed access to arginines for methylation by PRMTs. Our study revealed a novel role of PADI4 as a promoter-dependent epigenetic cofactor of Tal1, which interplays with important epigenetic histone marks and is accessible to pharmacological manipulation. Biotin purification and mass spectrometry Cells expressing the birA-Tal1 protein were grown in heavy (H) SILAC medium and control cells expressing the birA-ligase only, were grown in light SILAC medium (L) (RPMI SILAC medium, Thermo Scientific, Rockford, USA). For biotin purification of bir-Tal1, we used nuclear extracts of 1 × 10 8 K562-BirA control and K562-BirA-Tal1 cells [10] . Extracts were essentially prepared as described [63] . Biotinylated Tal1 was pulled out from cell extracts using streptavidin beads (Dynabeads M-280, Life Technologies, Oslo, Norway) and the beads were washed five times. As a control a pulldown from cells expressing only the birA-ligase was performed. BirA-Tal1 and the birA-ligase control samples were combined. Proteins were separated by one-dimensional SDS-PAGE (4–12% NuPAGE Bis-Tris Gel, Invitrogen) and the entire lane of the Coomassie blue-stained gel was cut into 23 slices. All slices were reduced with 10 mM dithiothreitol (DTT) for 55 min at 56 °C, alkylated with 55 mM iodoacetamide (IAA) for 20 min at 26 °C and digested with trypsin (Serva) overnight at 37 °C. Tryptic peptides were injected into a C18 precolumn (2.5 cm, 360 μm o.d., 100 μm i.d., Reprosil-Pur 120 Å, 5 μm, C18-AQ, Dr Maisch GmbH) at a flow rate of 10 μl min −1 . Bound peptides were eluted and separated on a C18 capillary column (20 cm, 360 μm o.d., 75 μm i.d., Reprosil-Pur 120 Å, 3 μm, C18-AQ, Dr Maisch GmbH) at a flow rate of 300 nl min −1 , with a gradient from 5 to 35% acetonitrile (ACN) in 0.1% formic acid for 90 min using an proxeon-nano-LC coupled to an Q-exactive mass spectrometer (Thermo Electron). Mass spectrometry (MS) conditions were as follows: spray voltage, 1.8 kV; heated capillary temperature, 270 °C; normalized collision energy 28. An underfill ratio of 1.2% and intensity threshold of 4.0 e4 were used. The mass spectrometer was operated in the data-dependent mode to automatically switch between MS and MS/MS acquisition. Survey MS spectra were acquired in the Orbitrap ( m / z 350–1,600) with the resolution set to 70,000 at m / z 200 and automatic gain control target at 2 × e 5 . The 15 most intense ions were sequentially isolated for higher-energy collisional dissociation MS/MS fragmentation and detection. Ions with single and unrecognized charge states were excluded. Raw data were analysed with ‘MaxQuant’ software (version 1.3.0.5). Uniprot human (version 27.08.2012 with 86,725 entries) was used as a sequence database. Up to two missed cleavages of trypsin were allowed. Oxidized methionine was searched as variable modifications, whereas cysteine carbamido-methylation as a fixed modification. The modifications corresponding to arginine and lysine labelled with heavy stable isotopes were handled as fixed modifications in the Maxquant search, if applicable, after identification of SILAC pairs by MaxQuant. The false-positive rate was set to 1% at the peptide level, the false discovery rate was set to 1% at the protein level and the minimum required peptide length was set to six amino acids. Proteins with an H/L ratio of >5 were defined as high-confidence members of the Tal1 interactome. The full list of identified proteins is given in Supplementary Data 1 . Interaction assays For endogenous CoIP 5 × 10 6 HEL cells were lysed in 500 μl IP-buffer buffer (50 mM Tris pH 7.5, 150 mM NaCl, 2 mM EDTA, 1% NP-40, 0.5% sodium deoxycholate, 5% glycerol and proteinase inhibitor cocktail) for 30 min at 4 °C on a rotating wheel. Lysates were centrifuged at 15,000 g for 30 min and the supernatants were divided into 100-μl aliquots. For CoIP, 200 μl of IP-buffer was added to each 100-μl aliquot. Three microgram of Tal1 antibody (Abcam, ab75738) or immunoglobulin (Ig)-G isotype control antibody (Santa-Cruz, sc-2027) and magnetic protein-G beads (Dynabeads protein-G beads, Life Technologies) were added. Upon incubation overnight at 4 °C on a rotating wheel, the beads were washed three times with IP-buffer and subjected to SDS-PAGE. Detection of immunoprecipitated Tal1 and coimmunoprecipitated PADI4 was performed by western blot using a PADI4 antibody (ab128086, Abcam 4H5, 1:2,000 dilution) and a Tal1 antibody (04–123, Millipore, BTL73, 1:500 dilution), respectively. For CoIP from HEK293 cells we used 3 × 10 4 HEK293 cells transfected with metafectene (Biontex). CoIP was performed as detailed [60] . Briefly, transiently transfected HEK293 cells were lysed in lysis buffer (50 mM Tris, pH 7.5, 100 mM NaCl, 0.1% Triton X-100, 1 mM DTT, 1 mM EDTA, 10% glycerol and protease inhibitors). After centrifugation the supernatant was collected and incubated with 10 μl of anti-FLAG agarose beads (M2, Sigma) at 4 °C for 4 h with rotation. The beads were washed four times with lysis buffer and the beads were resuspended in SDS-loading dye. The CoIP samples were analysed by western blot using an anti-HA antibody for detection of HA-PADI4 (sc-805, Santa-Cruz, 1:1,000) and anti-Tal1 antibody for the detection of Flag-Tal1 (sc-12984, Santa Cruz, 1:1,000 dilution). GST pull-down assays were performed as described [64] . Briefly, GST fusion proteins were expressed in E. coli (strain BL21). The GST protein was purified from lysates prepared in pull-down buffer (50 mM Tris, pH 7.5, 150 mM NaCl, 1 mM EDTA, 10% glycerol and 0.01% Nonidet P-40) using glutathione-agarose beads (Sigma-Aldrich). 35 S-labelled proteins were produced by coupled in vitro transcription/translation in the presence of [ 35 S]Met using the reticulocyte TNT-kit (Promega). The GST fusion protein was immobilized on glutathione-agarose beads and incubated with 10 μl of TNT reaction mixture in 300 μl of pull-down buffer at 4 °C for 1 h. The beads were washed four times using pull-down buffer. Upon elution of the proteins by boiling in SDS-loading-dye the samples were subjected to SDS-PAGE. Equal loading was assured by coomassie staining. Subsequently, the gel was dried, exposed to an X-ray film and analysed after 48 h. ChIP ChIP assays were performed in at least two independent experiments according to the Abcam-X-ChIP protocol with modifications [60] . For immunoprecipitation, the following antibodies were used: H3R2me2a (#07–585, Millipore, 4 μg) and H3K4me3 (ab1012, Abcam, 4 μg). H3K9Ac (ab10812, Abcam, 2 μg), H4R3me2a (39705, Active Motif, 4 μg), H3 (ab1791, Abcam, 3 μg), H3R17me2a (ab8284, Abcam, 4 μg), PRMT4/CARM1 (09–818, Millipore, 4 μg), Tal1 (ab75739, Abcam, 5 μg) and PADI4 (ab96758 in Figs 6 and 7 and ab128086 in Figs 4 and 5 , Abcam, 5 μg). The following IgGs were used as controls: IgG goat (Santa-Cruz, sc-2028), IgG mouse (Santa-Cruz, sc-2025) and IgG rabbit (Santa-Cruz, sc-2027). Purification of ChIP-DNA was performed using DNA purification columns (ChIP DNA Clean and Concentrator, Zymo Research, USA). ChIP-DNA was eluted with 40 μl of buffer and analysed by quantitative PCR using 2 μl of chromatin. Primer pairs are given in ( Supplementary Table 2 ). DNA recovery calculated as percent of the input, error bars represent the s.d. from at least four determinations. All ChIP data were confirmed with at least two independent chromatin preparations. Histone modification ChIP values were corrected for nucleosome density using values gathered with a Histone 3 ChIP. For ChIP-ReChIP, we diluted 70 μl of ChIP lysate with 210 μl RIPA buffer without SDS (50 mM Tris–HCl pH 7.5, 150 mM NaCl, 2 mM EDTA pH 8, 1% NP-40 and 0.5% sodium deoxycholate). In the first round of ChIP, two samples per antibody were prepared. Four micrograms was used for each antibody and 15 μl of magnetic protein-G beads (Life Technologies). Incubation was performed overnight at 4 °C on a rotating wheel. Subsequently, the beads were washed four times with wash buffer (20 mM Tris–HCl pH 7.5, 150 mM NaCl, 2 mM EDTA pH 8 and 1% Triton X-100) and eluted in 50 μl elution buffer-1 (50 mM Tris–HCl pH 7.5, 1% SDS and 15 mM DTT). At this stage the two samples were pooled and 700 μl of incubation buffer was added (50 mM Tris–HCl pH 7.5, 150 mM NaCl, 1% NP-40 and 0.25% sodium deoxycholate). For the second ChIP, 3 μg of antibody was added and incubated overnight at 4 °C. Upon elution of the DNA with elution buffer-2 (1% SDS and 100 mM NaCO 3 ) the sample was incubated with proteinase K, decross-linked at 65 °C and column purified as described for standard ChIP. P -values were calculated by an unpaired t -test (* P -value<0.05, ** P -value<0.01 and *** P -value<0.001). Cell culture K562 and HEL cells were obtained from ATCC and maintained in RPMI medium supplemented with 10% fetal calf serum, 1% penicillin/streptomycin and 1% glutamine. Lentiviral packaging was performed using HEK293T cells. HEL cells were at a cell density of 1.4 × 10 6 cells per well in a six-well plate. Transduction was performed with a multiplicity of infection of 100 and 8 μg ml −1 protamin sulphate. Human primary CD34+ cells from granulocyte colony-stimulating factor (G-CSF)-mobilized apheresis samples from healthy volunteer donors, with written informed consent and approval by the Ethics Committee (permit #329-10), were immunomagnetically enriched according to the manufacturer’s instructions (Miltenyi Biotech, Bergisch-Gladbach, Germany). Experiments were performed with CD34+ cells from at least two independent donors. hCD34+ cells were expanded for 3 days, transduced and sorted according to their green fluorescent protein signal. Subsequently, the transduced cells were seeded in MethoCult (Stem Cell Technologies, Grenoble, France). Colonies were evaluated 2 weeks after seeding, Supplementary Fig. 8 . The CD34+ cell isolation was controlled by flow cytometry using an anti-CD34 antibody (anti-CD34 pacific blue, Biolegend, Germany). Positive-selected cells were directly used or cryopreserved using CryoStor CS10 (Stem Cell Technologies) until further usage. Cells were expanded for 4 days at a cell density of 400,000–500,000 cells per millilitre in serum-free expansion medium (SFEM, Stem Cell Technologies) with cytokines (100 ng ml −1 FLT3, 100 ng ml −1 stem cell factor (SCF), 20 ng ml −1 IL-3 and 20 ng ml −1 IL-6). The cells were subjected to megakaryocytic (SFEM with 1 ng ml −1 SCF, 30 ng ml −1 thrombopoietin (TPO), 13.5 ng ml −1 IL-9 and 7.5 ng ml −1 IL-6) or erythrocytic differentiation (SFEM with 20 ng ml −1 SCF, 5 ng ml −1 IL-3, 2 μM dexamethasone, 0.2 μM estradiol and 1 U ml −1 erythropoietin (EPO)) for 6 days and used for mRNA analysis or ChIP. The efficiency of differentiation was controlled by flow cytometry using an CD41 or GYPA (GPA) antibody, respectively. Furthermore, quantitative reverse transcriptase-PCR with primers for beta-globin and CD41 were used to monitor erythrocytic and megakaryocytic differentiation. For monocytic differentiation, CD34+ cells were grown in monocytic differentiation medium (iscove's modified dulbecco's medium (IMDM) with 20% fetal calf serum, 30 ng ml −1 SCF, 30 ng ml −1 FLT-3, 30 ng ml −1 IL-3 and 30 ng ml −1 macrophage colony-stimulating factor (M-CSF)). Monocytic cells were isolated by CD14 magnetic microbeads (Miltenyi Biotech) to a purity of 95%. The efficiency was controlled by flow cytometry using an anti-CD14 antibody (anti-CD14 APC, Miltenyi Biotech). See also Supplementary Fig. 9 . Knockdown constructs ShRNA oligos against human PADI4 and human Tal1 were designed using the InvivoGen siRNAWizard program ( http://www.sirnawizard.com/design.php ) and cloned into a lentiviral backbone [60] . A non-specific shRNA was used as a control. Sequences targeted by shRNAs were: control-sh 5′-GACAAGAAACTAAGCAAGAAT-3′; shPADI4 5′-GCGAAGACCTGCAGGACAT-3′; 5′-GCCAACCAGAGCTGTGAAAGAT-3′; shTal1 5′-GACAAGAAGCTCAGCAAGAAT-3′; 5′-AAAGTTGTGCGGCGTATCTTC-3′. Cl-amidine The PADI4 inhibitor Cl-amidine was synthesized according to the slightly modified procedure described by Knuckley et al. [65] , or obtained commercially (Merck, Darmstadt, Germany). Step 1: ( S )-2-benzamido-5-(( tert -butoxycarbonyl)amino)pentanoic acid: ( S )-2-amino-5-(( tert butoxycarbonyl) amino)pentanoic acid (0.93 g, 4.0 mmol) was dissolved in a biphasic mixture of aqueous 3.5 M NaOH (1.2 ml) and Et2O (4 ml). The mixture was cooled to 0 °C and alternating portions of benzoyl chloride (0.46 ml, 4.0 mmol) and aqueous 8.5 M NaOH (4.0 mmol, 0.46 ml) were added every 5 min for 30 min. The reaction mixture was allowed to warm to room temperature and stirred overnight. The reaction was acidified (pH 1) with concentrated HCl and extracted with DCM (3 × 20 ml). The organics were combined, washed with brine, dried over MgSO 4 and concentrated to afford the product as a white powder (89% yield). Step 2: ( S )- tert- butyl (5-amino-4-benzamido-5-oxopentyl)carbamate: ( S )-2-benzamido-5-(( tert butoxycarbonyl) amino)pentanoic acid (2) (0.50 g, 1.5 mmol), HOTT ( S -(1-oxido-2-pyridinyl )-1,1,3,3-tetra-methylthiouronium hexafluorophosphate) (0.82 g, 2.23 mmol) and DIPEA ( N , N -diisopropylethylamine) (0.52 ml, 2.97 mmol) in DMF ( N , N -dimethylformamide) (5 ml). After stirring for 10 min, ammonium chloride (0.159 g, 2.97 mmol) was added and stirring continued for 45 min. The reaction was partitioned between EtOAc (ethylacetate) (25 ml) and brine (60 ml). The organics were combined and washed with 2 N HCl (2 × 12 ml), water (2 × 12 ml), saturated NaHCO 3 (2 × 12 ml), water (3 × 12 ml) and brine 12 ml. The organics were then dried over MgSO 4 and concentrated to afford the product as a white powder (92% yield). Step 3: ( S )- N -(1,5-diamino-1-oxopentan-2-yl)benzamide: ( S )- tert -butyl (5-amino-4-benzamido-5-oxopentyl)carbamate (3) (0.2 g, 0.60 mmol) was dissolved in cold trifluoroacetic acid (TFA) (6 ml) and stirred for 0 °C for 45 min. After warming to room temperature, TFA was removed under reduced pressure and the residue dissolved in water (5 ml) and washed with Et2O (5 ml) before being lyophilized (96% yield). Step 4: Ethyl 2-chloroacetimidate hydrochloride: in a 100-ml three-neck round-bottomed flask was 2-chloroacetonitrile (4.2 ml, 66.1 mmol) dissolved in EtOH (4.25 ml, 72.8 mmol) and Et2O (50 ml) to give a colourless solution. The mixture was cooled in an acetone/ice bath to −10 °C and HCl (g) was bubbled through the reaction. The temperature rose to 0 °C and HCl (g) was continuously bubbled (1 h). A white precipitate is formed and collected by filtration and rinsed with cold ether. A white solid is obtained (77% yield). Step 5: ( S )- N -(1-amino-5-(2-chloroacetimidamido)-1-oxopentan-2-yl)benzamide (Cl-amidine): ( S )- N -(1,5-diamino-1-oxopentan-2-yl)benzamide-TFA salt (0.194 g, 0,630 mmol) and triethylamine (0.26 ml, 1.89 mmol) were dissolved in MeOH (2 ml). Ethyl 2-chloroacetimidate hydrochloride (0.2 g, 1.26 mmol) was added and the mixture stirred overnight. The reaction mixture was quenched with water (5 ml) and acidified with TFA. The product was isolated by preparative HPLC-MS using an isocratic method (18% MeOH, 0.1% formic acid and water) as a white powder (5% yield). See also Supplementary Fig. 10 . Gene expression analysis Total RNA was isolated using the RNeasy mini kit (Qiagen, Hilden, Germany). Complementary DNA (cDNA) was synthesized using the Omniscript reverse transcriptase (Qiagen). Quantitative PCR was performed on a LightCycler 480 (Roche, Mannheim, Germany) using SYBR-Green PCR MasterMix (Eurogentec, Liege Belgium). Values were normalized against glyceraldehyde 3-phosphate dehydrogenase expression. Error bars represent the s.d. of at least four independent evaluations. Primer sequences are given in Supplementary Table 3 . Microarray analysis and data analysis Gene expression array analysis of shTal1 and shPADI4 HEL cells was done with a whole-genome 4 × 44K gene array (GPL13497, Agilent Technologies, Santa Clara, CA, USA). Array analysis was performed in triplicate. Microarrays were done using the ‘Low RNA Input linear Amplification Kit Plus, One Color’ protocol (Agilent Technologies) and the Agilent RNA Spike-In Kit for One color (Agilent Technologies) following the manufacturer’s standard protocol. Total RNA (200 ng) were used as a starting material to prepare cDNA. cDNA synthesis and in vitro transcription were performed according to the manufacturer’s recommendation. Quantity and efficiency of the labelled amplified cDNA were determined using the NanoDrop ND-1000 UV–vis Spectrophotometer version 3.2.1. The hybridizations were performed for 17 h at 10 r.p.m. and 65 °C in the Hybridization Oven (Agilent Technologies). Washing and staining of the arrays were done according to the manufacturer’s recommendation. Cy3 intensities were detected by one-colour scanning using an Agilent DNA microarray scanner. Scanned image files were visually inspected for artifacts and then analysed [66] . Intensity data were extracted using Agilent’s Feature Extraction software (version 11.5.1.1) including a quality control based on internal controls using Agilent’s protocol GE1_107_Sep09. All chips passed the quality control and were analszed using the Limma package [67] of Bioconductor [68] . Candidate genes were filtered to a minimum of twofold change and false discovery rate-corrected P -value <0.05. For functional characterization of the differentially expressed transcripts, GO enrichment analysis was conducted via goseq accounting for gene length bias and correcting for multiple testing. Further functional association of candidate genes was performed with the webtool DAVID. Mutagenesis Mutagenesis of PADI4 was performed using site-directed mutagenesis. The inactive PADI4 double-mutant R374A/C645A was constructed according to published data [49] , [69] ( Supplementary Fig. 2 ). Sequencing validated the integrity of wild-type and mutant PADI4. Expression and activity of mutant PADI4 was tested by enzymatic assay and western blot with transfected PADI4 and PADI4 mutant ( Supplementary Fig. 11 ). Immunoblotting and FACS Immunoblot analysis was performed using anti-Tal1 (sc-12984, Santa-Cruz, 1:1,000 dilution and 04–123, Millipore, 1:500 dilution), anti-PADI4 (ab96758, 1:500 dilution and ab128086, 1:2,000 dilution, Abcam), anti-HA (sc-805, Santa-Cruz, 1:1,000 dilution), anti-Flag (F3165, 1:4,000 dilution, Sigma-Aldrich), anti-LaminB1 (ab16048, Abcam, 1:1,000 dilution) and anti-CTCF (ab70303, Abcam, 1:1,000 dilution). Western blots were analysed using X-ray film or an imaging system (Fusion FX7, PEQLAB, Erlangen, Germany). Uncropped images are provided in Supplementary Figs 12–15 . FACS analysis of gp130 surface staining was performed using an APC-labelled gp130 antibody (R&D Systems, FAB228A). Accession Codes : Microarray data have been deposited in NCBI’s Gene Expression Omnibus under accession number GSE54075 . How to cite this article: Kolodziej, S. et al. PADI4 acts as a coactivator of Tal1 by counteracting repressive histone arginine methylation. Nat. Commun. 5:3995 doi: 10.1038/ncomms4995 (2014).